Structural basis for preferential avian receptor binding by the human-infecting H10N8 avian influenza virus Since December 2013, at least three cases of human infections with H10N8 avian influenza virus have been reported in China, two of them being fatal. To investigate the epidemic potential of H10N8 viruses, we examined the receptor binding property of the first human isolate, A/Jiangxi-Donghu/346/2013 (JD-H10N8), and determined the structures of its haemagglutinin (HA) in complex with both avian and human receptor analogues. Our results suggest that JD-H10N8 preferentially binds the avian receptor and that residue R137—localized within the receptor-binding site of HA—plays a key role in this preferential binding. Compared with the H7N9 avian influenza viruses, JD-H10N8 did not exhibit the enhanced binding to human receptors observed with the prevalent H7N9 virus isolate Anhui-1, but resembled the receptor binding activity of the early-outbreak H7N9 isolate (Shanghai-1). We conclude that the H10N8 virus is a typical avian influenza virus. Influenza A virus is a major threat to public health—causing seasonal flu and occasional pandemics—with extensive attention paid to the recently identified human-infecting avian influenza A viruses [1] , [2] , [3] , [4] . Different subtypes of avian influenza A viruses have caused sporadic human infections in the past, including H5N1, H6N1, H7N9 and H9N2 (refs 1 , 2 , 5 , 6 , 7 , 8 , 9 , 10 ). Since the first human infection with avian influenza A (H5N1) virus was reported in Hong Kong in 1997 (refs 5 , 6 ), the H5N1 virus has caused more than 600 cases of human infections, with a fatality rate of ~60% ( http://www.who.int/influenza/human_animal_interface/H5N1_cumulative_table_archives/en/ ). The influenza A H7N9 virus was first identified in China in 2013 and has caused more than 400 cases of human infections, with a fatality rate of ~30% ( http://www.who.int/influenza/human_animal_interface/influenza_h7n9/en/ ). Since December 2013, at least three new cases of human infections with the avian H10N8 subtype virus have been reported, and two of the infected individuals died [11] . Exploring the epidemic potential of this H10N8 virus is crucial for the development of effective preventive and therapeutic measures. Here we evaluate this strain’s receptor-binding properties and the molecular basis for its activity. Using solid-phase binding assay, surface plasmon resonance (SPR) and tissue staining, we find that the H10N8 virus preferentially binds the avian receptor with negligible binding to the human receptor. Crystal structures of H10 protein in complex with avian or human receptor analogues reveal that residue R137, located in the receptor-binding site of HA, plays a key role in the preferential binding to the avian receptor. Receptor-binding property of H10N8 The receptor binding activity of influenza virus is thought to be a major determinant of virus transmissibility, which is determined by the viral surface glycoprotein HA [12] , [13] , [14] . To characterize the receptor-binding activity of the human-infecting H10N8 virus, we rescued the human isolate A/Jiangxi-Donghu/346/2013 (JD-H10N8) using reverse genetics technology, naming the rescued virus rJD-H10N8. We analyzed the receptor-binding properties of rJD-H10N8 through solid-phase binding assays in comparison with two H7N9 virus isolates simultaneously (A/Shanghai/1/2013, SH-H7N9, isolated from only a few patients; and A/Anhui/1/2013, AH-H7N9, the prevalent isolate in both the 2013 and 2014 outbreaks in China), a pandemic virus isolate (A/California/04/2009 (H1N1), CA04-H1N1) and a typical avian influenza virus isolate (A/Anhui/1/2005 (H5N1), AH05-H5N1). We find that JD-H10N8 preferentially bound the avian receptor, with limited binding to the human receptor ( Fig. 1a ), which is similar to the SH-H7N9 virus ( Fig. 1b ), the early isolate of the 2013 outbreak in China. In contrast, AH-H7N9 preferentially bound the avian receptor, but also exhibited high affinity to the human receptor ( Fig. 1c ) [15] . As controls, the human influenza virus CA04-H1N1 preferentially bound the human receptor ( Fig. 1d ) and the avian influenza virus AH05-H5N1 preferentially bound the avian receptor ( Fig. 1e ). These data demonstrate that the JD-H10N8 virus has similar receptor-binding properties to the early H7N9 isolate of SH-H7N9 (Shanghai-1) and remains an avian virus with the potential for sporadic human infections. 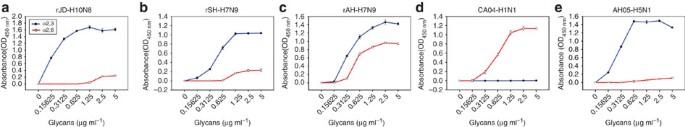Figure 1: Receptor-binding properties at the virus level. Solid-phase binding assays for (a) rJD-H10N8 (reverse genetics-rescued JD-H10N8), (b) rSH-H7N9 (reverse genetics-rescued A/Shanghai/1/2013), (c) rAH-H7N9 (reverse genetics-rescued A/Anhui/1/2013), (d) CA04-H1N1 (A/California/04/2009) and (e) AH05-H5N1 (A/Anhui/1/2005) viruses to both α2,3-linked (3′SLNLN) or α2,6-linked sialylglycan receptors (6′SLNLN). Binding to 3′SLNLN is coloured in blue and 6′SLNLN in red. JD-H10N8 preferentially binds to 3′SLNLN. As a comparison, rSH-H7N9 binds preferentially to 3′SLNLN such as JD-H10N8, while rAH-H7N9 binds both 3′SLNLN and 6′SLNLN. As a control, CA04-H1N1 specifically binds 6′SLNLN and AH05-H5N1 specifically binds 3′SLNLN. Error bars represent s.d. of the mean, which is calculated with three independent repeats. Figure 1: Receptor-binding properties at the virus level. Solid-phase binding assays for ( a ) rJD-H10N8 (reverse genetics-rescued JD-H10N8), ( b ) rSH-H7N9 (reverse genetics-rescued A/Shanghai/1/2013), ( c ) rAH-H7N9 (reverse genetics-rescued A/Anhui/1/2013), ( d ) CA04-H1N1 (A/California/04/2009) and ( e ) AH05-H5N1 (A/Anhui/1/2005) viruses to both α2,3-linked (3′SLNLN) or α2,6-linked sialylglycan receptors (6′SLNLN). Binding to 3′SLNLN is coloured in blue and 6′SLNLN in red. JD-H10N8 preferentially binds to 3′SLNLN. As a comparison, rSH-H7N9 binds preferentially to 3′SLNLN such as JD-H10N8, while rAH-H7N9 binds both 3′SLNLN and 6′SLNLN. As a control, CA04-H1N1 specifically binds 6′SLNLN and AH05-H5N1 specifically binds 3′SLNLN. Error bars represent s.d. of the mean, which is calculated with three independent repeats. Full size image To further evaluate the receptor-binding affinities of JD-H10N8 for canonical avian and human receptor analogues, we generated soluble HA protein from JD-H10N8 using a baculovirus expression system [16] , [17] . Using SPR, we found that JD-H10N8 HA bound the avian receptor analogue with an affinity of 0.4 μM ( Fig. 2a ). By contrast, the JD-H10N8 HA had extremely weak binding to the human receptor ( K D >1 mM, beyond the SPR measurement range, Fig. 2a ). This binding activity is very similar to that of the A/Shanghai/1/2013(H7N9) hemagglutinin (SH-H7N9 HA) protein but distinct to that of the A/Anhui/1/2013(H7N9) hemagglutinin (AH-H7N9 HA) protein [15] . SH-H7N9 HA also exhibited binding preference towards the avian receptor—with a similarly high affinity of 0.16 μM and extremely weak binding to the human receptor ( Fig. 2b )—whereas AH-H7N9 HA bound both avian and human receptors with high affinities (0.10 and 0.33 μM, respectively, Fig. 2c ). As controls, A/California/04/2009 (H1N1) hemagglutinin (CA04-H1N1 HA) is shown to preferentially bind the human receptor analogue and A/Anhui/1/2005(H5N1) (AH05-H5N1) HA to bind the avian receptor ( Fig. 2d,e ). Collectively, the soluble HA-binding experiments yielded results similar to the above whole virus binding data. 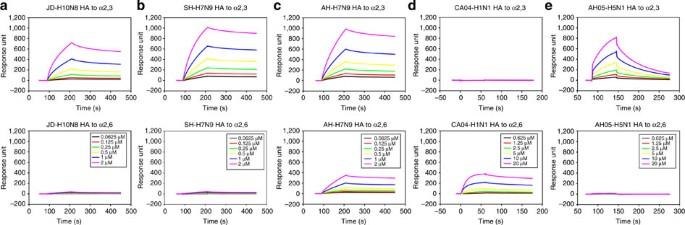Figure 2: Receptor-binding properties at the protein level. BIAcore diagrams showing binding of JD-H10N8 HA to 3′SLNLN and 6′SLNLN (a), SH-H7N9 HA to 3′SLNLN and 6′SLNLN (b), AH-H7N9 HA to 3′SLNLN and 6′SLNLN (c), CA04-H1N1 HA to 3′SLNLN and 6′SLNLN (d), and AH05-H5N1 HA to 3′SLNLN and 6′SLNLN (e). Similar to the receptor-binding properties at the virus level, JD-H10N8 HA and SH-H7N9 HA preferentially bind 3′SLNLN, while AH-H7N9 HA binds both 3′SLNLN and 6′SLNLN. As controls, CA04-H1N1 HA preferentially binds 6′SLNLN and AH05-H5N1 HA preferentially binds 3′SLNLN. Figure 2: Receptor-binding properties at the protein level. BIAcore diagrams showing binding of JD-H10N8 HA to 3′SLNLN and 6′SLNLN ( a ), SH-H7N9 HA to 3′SLNLN and 6′SLNLN ( b ), AH-H7N9 HA to 3′SLNLN and 6′SLNLN ( c ), CA04-H1N1 HA to 3′SLNLN and 6′SLNLN ( d ), and AH05-H5N1 HA to 3′SLNLN and 6′SLNLN ( e ). Similar to the receptor-binding properties at the virus level, JD-H10N8 HA and SH-H7N9 HA preferentially bind 3′SLNLN, while AH-H7N9 HA binds both 3′SLNLN and 6′SLNLN. As controls, CA04-H1N1 HA preferentially binds 6′SLNLN and AH05-H5N1 HA preferentially binds 3′SLNLN. Full size image Host tissue tropism of H10N8 To examine the host tissue tropism of JD-H10N8 HA, we used soluble recombinant HA protein to stain paraffinized human trachea and duck intestinal tract sections. It is known that through lectin staining, the apical surface of the human trachea predominantly displays diverse glycan receptors terminated by α2,6 sialic acid linkages (human receptors) [18] , whereas the apical surface of the duck intestinal tract is full of diverse glycan receptors terminated by α2,3 sialic acid linkages (avian receptors) [19] . Consistent with the SPR experiments, JD-H10N8 HA did not stain the human trachea but stained the duck small intestine well ( Fig. 3 ). As a comparison, SH-H7N9 HA did not stain the human trachea but stained the duck small intestine like JD-H10N8 HA, whereas AH-H7N9 HA stained both the human trachea (with a low intensity) and the duck small intestine (strongly) ( Fig. 3 ). As controls, the HA from the human-adapted CA04-H1N1 virus could stain the human trachea well but could not stain the duck intestinal tract, whereas the HA from the avian AH05-H5N1 displayed the same host tropism as JD-H10N8 HA ( Fig. 3 ). These experiments further suggest that JD-H10N8 is a typical avian influenza virus. 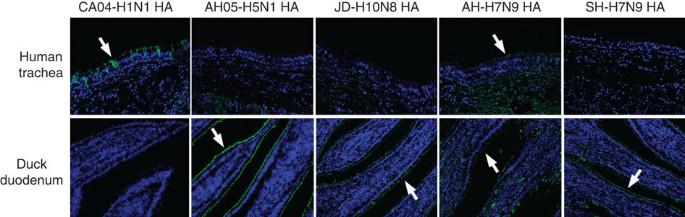Figure 3: Staining of human trachea and duck small intestine with JD-H10N8 HA and other HAs. Paraffinized tissue sections were stained with recombinant HAs derived from the baculovirus expression system. Specific staining by recombinant HA (in green) is indicated by white arrows. The apical surface of the human trachea is rich in α2,6-linked glycan receptors and the apical surface of the duck small intestine is full of α2,3-linked glycan receptors. JD-H10N8 HA and SH-H7N9 HA did not stain the human trachea but stained the duck small intestine. AH-H7N9 HA stained the duck small intestine and also stained the human trachea with low intensity. As controls, CA04-H1N1 HA stained the human trachea well without any staining of the duck small intestine, and AH05-H5N1 HA stained the duck small intestine well without any staining of the human trachea. Figure 3: Staining of human trachea and duck small intestine with JD-H10N8 HA and other HAs. Paraffinized tissue sections were stained with recombinant HAs derived from the baculovirus expression system. Specific staining by recombinant HA (in green) is indicated by white arrows. The apical surface of the human trachea is rich in α2,6-linked glycan receptors and the apical surface of the duck small intestine is full of α2,3-linked glycan receptors. JD-H10N8 HA and SH-H7N9 HA did not stain the human trachea but stained the duck small intestine. AH-H7N9 HA stained the duck small intestine and also stained the human trachea with low intensity. As controls, CA04-H1N1 HA stained the human trachea well without any staining of the duck small intestine, and AH05-H5N1 HA stained the duck small intestine well without any staining of the human trachea. Full size image Structural basis for preferential binding to the avian receptor Using X-ray crystallography, we determined the structures of JD-H10N8 in either its free form or in complex with the two sialo-pentasaccharides 3′SLNLN and 6′SLNLN. These sialo-pentasaccharides are analogues of the avian and human receptors, respectively, and contain the same three terminal saccharides (Sia-Gal-GlcNAc) [20] but with different glycosidic linkages (α2,3-linkage for the avian receptor and α2,6-linkage for the human receptor). With resolution for the structures of 2.5, 2.6 and 2.3 Å, respectively ( Table 1 ), clear electron densities are observed for the ligands in both complexes ( Fig. 4 ). Table 1 Statistics for crystallographic data collection and structure refinement. 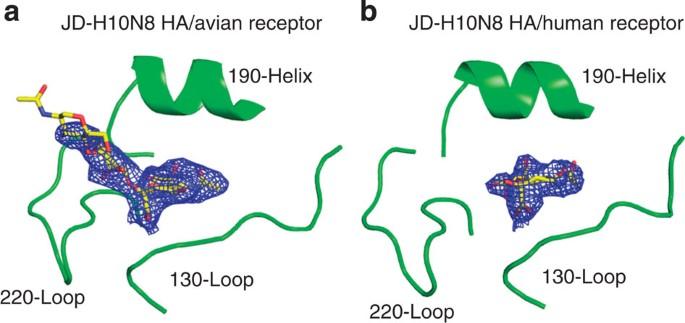Figure 4: 2Fo−Fcmaps for the glycan receptors in the JD-H10N8 HA/receptor complex structures. 2Fo−Fcmaps for the glycan receptors in the JD-H10N8 HA/receptor complex structures (a) JD-H10N8 HA/3′SLNLN and (b) JD-H10N8 HA/6′SLNLN. The panels show portions of 2Fo−Fcelectron density maps for these glycan receptor analogues contoured at 1.0σsigma and 0.8σ, respectively, and the figures were drawn by Pymol software. The 2Fo−Fcmaps were generated by FFT programme in CCP4 software. Full size table Figure 4: 2 F o − F c maps for the glycan receptors in the JD-H10N8 HA/receptor complex structures. 2 F o − F c maps for the glycan receptors in the JD-H10N8 HA/receptor complex structures ( a ) JD-H10N8 HA/3′SLNLN and ( b ) JD-H10N8 HA/6′SLNLN. The panels show portions of 2 F o − F c electron density maps for these glycan receptor analogues contoured at 1.0 σ sigma and 0.8 σ , respectively, and the figures were drawn by Pymol software. The 2 F o − F c maps were generated by FFT programme in CCP4 software. Full size image The structure of JD-H10N8 HA with the avian receptor analogue 3′SLNLN reveals that the analogue binds in a trans conformation ( Fig. 5a ). Three conserved hydrogen bonds are formed between the Sia-1 and the 130-loop residues (the main-chain carbonyl group of T135, the side-chain hydroxyl group of T136 and the main-chain amino group of residue R137), which have been observed in most of the HA–receptor complex structures. For the 220-loop, the hydrophilic residue Q226 directly forms two hydrogen bonds with the sialic acid (Sia-1) and a hydrogen bond network is formed between the Sia-1 and Q226 and G228, mediated by a water molecule. For the 190-helix, the residue E190 forms two hydrogen bonds with the Sia-1. All of the hydrogen bond interactions between the HA and receptor analogue are converged on the Sia-1. 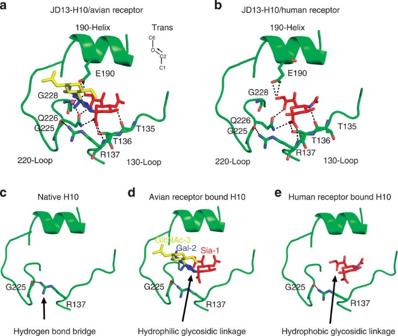Figure 5: Structural analyses of the interactions of JD-H10N8 HA with either avian or human receptor analogues. The three secondary structural elements of the binding site (that is, the 130-loop, 190-helix and 220-loop; H3 numbering) are labelled in ribbon representation, together with the selected residues in stick representation. The hydrogen bonds are shown as black dashed lines. JD-H10N8 HA with the avian receptor analogue (a) or human receptor analogue (b) bound. The avian receptor analogue binds in a typicaltransconformation, whereas only the sialic acid moiety is observed in the JD-H10N8 HA/human receptor analogue complex. In the native JD-H10N8 HA structure (c), residue R137 forms a potential hydrogen bond with the main-chain carbonyl oxygen atom of residue G225; this interaction is called a ‘hydrogen bond bridge’ here. In the JD-H10N8 HA/avian receptor analogue complex (d), the hydrogen bond bridge provides a favourable hydrophilic environment for the hydrophilic glycosidic linkage of the avian receptor analogue. In the JD-H10N8 HA/human receptor analogue complex (e), the hydrogen bond bridge provides an unfavourable hydrophilic environment for the hydrophobic glycosidic linkage of the human receptor analogue. Figure 5: Structural analyses of the interactions of JD-H10N8 HA with either avian or human receptor analogues. The three secondary structural elements of the binding site (that is, the 130-loop, 190-helix and 220-loop; H3 numbering) are labelled in ribbon representation, together with the selected residues in stick representation. The hydrogen bonds are shown as black dashed lines. JD-H10N8 HA with the avian receptor analogue ( a ) or human receptor analogue ( b ) bound. The avian receptor analogue binds in a typical trans conformation, whereas only the sialic acid moiety is observed in the JD-H10N8 HA/human receptor analogue complex. In the native JD-H10N8 HA structure ( c ), residue R137 forms a potential hydrogen bond with the main-chain carbonyl oxygen atom of residue G225; this interaction is called a ‘hydrogen bond bridge’ here. In the JD-H10N8 HA/avian receptor analogue complex ( d ), the hydrogen bond bridge provides a favourable hydrophilic environment for the hydrophilic glycosidic linkage of the avian receptor analogue. In the JD-H10N8 HA/human receptor analogue complex ( e ), the hydrogen bond bridge provides an unfavourable hydrophilic environment for the hydrophobic glycosidic linkage of the human receptor analogue. Full size image In the structure of JD-H10N8 HA in complex with the human receptor analogue 6′SLNLN, only the sialic acid moiety is observed ( Fig. 5b ), with a poor electron density map. Three conserved hydrogen bonds are formed between the Sia-1 and the 130-loop residues. For the 220-loop, the hydrophilic residue Q226 directly forms two hydrogen bonds with the Sia-1, but the hydrogen bond network that is observed in the JD-H10N8 HA/avian receptor complex structure cannot be observed, probably because of poor binding. For the 190 helix, the residue E190 forms two hydrogen bonds with the Sia-1. Further structural analyses reveal that R137 residue is important for receptor binding in JD-H10N8 HA. In the native JD-H10N8 structure ( Fig. 5c ), a hydrogen bond bridge is formed between the side chain of residue R137 and the main-chain carbonyl oxygen of G225, which has not been observed in other HA subtypes. In the JD-H10N8 HA/avian receptor complex structure ( Fig. 5d ), the side chain of residue R137 has no hydrogen bonds with the avian receptor analogue, and the hydrogen bond bridge provides a favourable hydrophilic environment for the exposed hydrophilic glycosidic linkage in the avian receptor analogue 3′SLNLN. In the JD-H10N8 HA–human receptor complex structure ( Fig. 5e ), the hydrogen bond bridge could create an unfavourable hydrophilic environment for the exposed hydrophobic glycosidic linkage of the human receptor. Alternatively, as R137 forms a hydrogen bond with the 220-loop, it may stabilize the loop so that it favours binding to the avian receptor more than the human receptor [21] , [22] . These could explain why the JD-H10N8 HA displays strong binding to avian receptor but very weak binding to the human receptor. To date, the H5N1, H7N9 and H10N8 avian influenza viruses have caused severe infection in humans, representing a health threat. Since 1997, the H5N1 viruses have caused more than 600 human infections in ~17 years, whereas for the H7N9 viruses that emerged in February 2013, more than 400 human infections have been reported in less than 2 years (ref. 23 ). The different outcomes could be due to the different receptor-binding properties of the H5N1 and H7N9 viruses [15] , [24] , [25] , [26] , [27] , [28] , [29] , [30] , [31] , [32] . The H5N1 viruses display strong binding to avian receptors and weak binding to human receptors, and sporadically infect humans. By contrast, the H7N9 viruses, with a dominant prevalent strain (Anhui-1), display preferential binding to avian receptors with increased binding to human receptors [15] . More importantly, the viruses in the first few reported cases—represented by the Shanghai-1 virus—predominantly bind to avian receptors but with very limited human receptor binding. Thus, for the first time, we have seen mutations of the avian virus with increased human receptor binding capability during an outbreak. In this study, we find that the receptor binding activity of the JD-H10N8 virus resemble the H5N1 and Shanghai-1 H7N9 avian influenza viruses by solid-phase binding assays with whole virus, as well as SPR experiments and tissue staining with isolated proteins. Our data suggest that the JD-H10N8 virus would probably not cause an epidemic similar to the H7N9 virus in its present form. However, surveillance should be emphasized for H10N8 in the event that it acquires new mutations in HA protein as seen for H7N9 between Shanghai-1 and Anhui-1. Recently, Skehel and colleagues [33] examined the receptor-binding properties of an avian H10N2 virus, revealing that the avian H10 virus possesses high avidity for human receptors. The lower avidities observed in our work might reflect the different methods used (for example, under different temperature settings). However, both reports observed affinity in similar millimolar (mM) range. In their avian H10/human receptor analogue complex structure, they observed that the residue Q222 of the 220 loop forms a strong hydrogen bond with the human receptor, which is used to explain the phenomenon that avian H10 virus has high avidity for human receptors. Then, based on the similarity of residues in the receptor-binding site of HAs between the avian H10 virus and human-infecting H10 virus, Vachieri et al. [33] concluded that the human-infecting H10 virus should possess a high avidity for human receptors. In their human-infecting H10/human receptor analogue complex structure, they observed that residue R137 forms a ‘potential’ hydrogen bond with the human receptor, which is helpful for human receptor binding [33] . Note that in avian H10, the residue at position 137 is a lysine (K), which points away from the receptor-binding site and has no hydrogen bond interaction with the human receptor, leading to a minimal impact on the 220-loop residues including Q222. However, our own structure of human-infecting H10 bound to human receptor R137 does not form a hydrogen bond with the human receptor, but instead forms a hydrogen bond with G225 in the 220 loop. Thus, we speculate that R137 might be flexible and able to adopt different conformations. Taken together, work from our and Skehel’s groups indicate that the H10 subtype preferentially binds the avian receptor, while the avian H10 with Lysine at position 137 possesses some human receptor-binding capacity, and the human-infecting H10 with an arginine at position 137 has a limited ability to bind the human receptor. Protein expression and purification The genes encoding the ectodomains of the HA from JD-H10N8 (JD-H10N8 HA) was cloned into the baculovirus transfer vector pFastBac1 (Invitrogen) in-frame with an amino-terminal gp67 signal peptide for secretion, a C-terminal thrombin cleavage site, a trimerization foldon sequence and a His 6 -tag at the extreme carboxy terminus for purification. Transfection and virus amplification were performed according to the Bac-to-Bac baculovirus expression system manual (Invitrogen) [15] , [16] , [17] . HAs of SH-H7N9 HA, AH-H7N9 HA, CA04-H1N1 HA and AH05-H5N1 HA were prepared as described in our previous report [15] . HA proteins were produced by infecting suspension cultures of Hi5 cells (Invitrogen) for 2 days. Soluble HAs were recovered from cell supernatants by metal affinity chromatography using a HisTrap HP 5-ml column (GE Healthcare), then purified by ion-exchange chromatography using a Mono-Q 4.6/100 PE column (GE Healthcare). The purified proteins were subjected to thrombin digestion (Sigma, 3 units per mg HA; overnight at 4 °C) to remove the C-terminal trimerization foldon sequence and His 6 -tag. For crystallization, the proteins were further purified by gel filtration chromatography using a Superdex-200 16/60 GL column (GE Healthcare) with a running buffer of 20 mM Tris–HCl and 50 mM NaCl (pH 8.0), and the collected protein fractions were concentrated to 8 mg ml −1 . Crystallization and structure determination H10 protein was crystallized via the sitting-drop vapour diffusion method at 18 °C. The H10 crystals grew in a reservoir solution of 15% w/v PEG 2000 MME, 0.1 M potassium chloride, 0.1 M Tris, pH 8.0. For receptor analogue complexes, crystals were soaked in a reservoir solution containing 10 mM 3′SLNLN (NeuAcα2-3Galβ1-4GlcNAcβ1-3Galβ1-4Glc) or 6′SLNLN (NeuAcα2-6Galβ1-4GlcNAcβ1-3Galβ1-4Glc) (kindly provided by the Consortium for Functional Glycomics (Department of Molecular Biology, Scripps Research Institute, La Jolla, CA)) for 4 h. All crystals were flash-cooled in liquid nitrogen after a brief soaking in reservoir solution with the addition of 17% (v/v) glycerol. The X-ray diffraction data were collected at Shanghai Synchrotron Radiation Facility beamline 17 U, with a wavelength of 1,000 angstrom, at a temperature of 100 K. All data were processed with HKL2000 software [34] . The H10 structures were solved by molecular replacement using Phaser [35] from the CCP4 programme suite [36] , with the structure of the H7N3 HA from A/TURKEY/ITALY/215845/2002 (PDB code: 4BSG) as a search model. The H10 and receptor analogue complexes were subsequently determined using the refined H10 structure as input model. Initial rigid body refinement was performed using REFMAC5 (ref. 37 ) and extensive model building was performed using COOT [38] . Further rounds of refinement were carried out using the phenix.refine programme implemented in the PHENIX package [39] with energy minimization, isotropic ADP refinement and bulk solvent modelling. The structures were then adjusted using COOT and refined with PHENIX. Final statistics for data collection and structure refinement are represented in Table 1 . The stereochemical quality of the final model was assessed with the programme PROCHECK [40] . The Ramachandran plot revealed that there is no atoms in the disallowed region, and ~90% of the atoms are in most favoured regions. SPR experiments The affinity and binding kinetics of HAs to receptor analogues were all analysed at 25 °C on a BIAcore 3000 machine with streptavidin chips (SA chips, GE Healthcare). PBS containing 0.005% Tween 20 (PBST) was used as the kinetics analysis buffer. Two biotinylated receptor analogues, the α-2,6 glycan (6′SLNLN: NeuAcα2-6Galβ1-4GlcNAcβ1-3Galβ1-4GlcNAcβ1-SpNH-LC-LC-Biotin) and the α-2,3 glycan (3′SLNLN: NeuAcα2-3Galβ1-4GlcNAcβ1-3Galβ1-4GlcNAcβ1-SpNH-LC-LC-Biotin) were kindly provided by the Consortium for Functional Glycomics (Department of Molecular Biology, Scripps Research Institute). Approximately 400 response units of biotinylated glycans were immobilized on the chip and a blank channel was used as the negative control. Thrombin-digested HAs were purified by gel filtration using PBST buffer as the running buffer and serially diluted to concentrations ranging from 0.0625 to 2 μM (JD-H10N8 HA, SH-H7N9 HA and AH-H7N9 HA) or from 0.625 to 20 μM (CA04-H1N1 HA and AH05-H5N1 HA). The HA protein preparations were then flowed through the chip and the response units were measured. The sensor surface was regenerated with 10 mM NaOH at the end of each cycle. Sensograms were globally fitted with BIAcore 3000 analysis software (BIAevaluation Version 4.1) using a 1:1 Langmuir binding mode and HA monomer as the identity to assume a 1:1 binding. The affinity values were calculated with a simultaneous kinetic K a (association rate)/ K d (dissociation rate) model. Binding of HAs to human and duck tissue sections The immunofluorescence assay was based on those reported by Chandrasekaran et al. [41] and Tharakaraman et al. [42] Briefly, paraffinized human tracheal and duck small intestine tissue sections were deparaffinized, rehydrated and incubated with 1% BSA in PBS for 30 min at room temperature (RT) to prevent nonspecific binding. Ion-exchange chromatography-purified HA (still with trimerization foldon sequence and His 6 -tag) was precomplexed with primary antibody (mouse anti-His-tag, MBL) and secondary antibody (Alexa Fluor 488 goat anti-mouse IgG, Invitrogen) in a molar ratio of 4:2:1, respectively, for 20 min on ice. The tissue binding was performed using HA concentration (50 μg ml −1 ) by diluting the precomplexed stock HA in 1% BSA–PBS. Tissue sections were then incubated with the HA–antibody complexes for 3 h at RT. Sections were counterstained with DAPI (Beyotime; 1:1,000 in PBS) for nuclei for 20 min at RT. After thorough washing, the tissue sections were mounted and then examined by using confocal laser scanning microscopy (Leica TCS SP8 laser scanning confocal microscopy). Virus preparations The experiments were performed in the approved Biosafety level 3 laboratory. The A/Anhui/1/2013 (AH-H7N9) and A/Shanghai/1/2013 (SH-H7N9) viruses were generated by plasmid-based reverse genetics technology to avoid any impurities of the initial isolated viruses as previously described [15] . The rescued viruses were named rAH-H7N9 and rSH-H7N9, respectively, to distinguish from the natural isolates. A re-assortant JD-H10N8 (rJD-H10N8) virus was also rescued by plasmid-based reverse genetics technology [43] . The rJD-H10N8 virus comprised H10 HA and N8 NA from JD-H10N8 virus, and the remaining six gene segments are derived from PR8/H1N1 virus. All rescued viruses were sequenced to exclude any unwanted mutations. The CA04-H1N1 and AH05-H5N1 are original virus isolates stocked in our laboratory. Virus stocks were propagated in specific pathogen-free chicken embryonated eggs. Virus concentrations were determined by using haemagglutination (HA) assays with 1% (vol/vol) chicken red blood cells. Solid-phase binding assay Receptor-binding specificity was analysed by a solid-phase direct binding assay [44] . Briefly, Serial dilutions (0.15625, 0.3125, 0.625, 1.25, 2.5 and 5 μg ml −1 ) of biotinylated glycans 3′SLNLN and 6′SLNLN were prepared in PBS, and 50 μl was added to the wells of the streptavidin-coated high binding capacity 96-well plate (Pierce) and allowed to attach overnight at 4 °C. After removal of the glycopolymer solution, the plates were blocked with 100 μl of PBS containing 2% BSA at RT for 1 h. After washing with ice-cold PBS containing 0.1% Tween 20 (PBST), the plates were incubated in a solution containing influenza virus (256 HA units in PBST), 10 μM oseltamivir and 10 μM zanamivir at 4 °C for 12 h. After washing with PBST, rabbit antisera (against JD-H10N8 HA, CA04-H1N1 HA, AH05-H5N1 HA or AH-H7N9 HA, respectively) was added to each well and the plates were incubated at 4 °C for 5 h. The wells were then washed with ice-cold PBST and incubated with horseradish peroxidase-conjugated goat-anti-rabbit IgG (Santa Cruz Biotechnology) for 2 h at 4 °C. After washing with ice-cold PBST, the plates were incubated with 100 μl TMB Horseradish Peroxidase Color Development Solution (Beyotime) for 10 min at RT. The reaction was stopped with 50 μl of 1 M H 2 SO 4 and the absorbance was determined at 450 nm. Accession codes: The structures for JD-H10N8 HA, JD-H10N8 HA/3′SLNLN and JD-H10N8 HA/6′SLNLN are deposited to Protein Data Bank with the accession numbers, 4QY0 , 4QY1 and 4QY2 , respectively. How to cite this article: Wang, M. et al. Structural basis for preferential avian receptor binding by the human-infecting H10N8 avian influenza virus. Nat. Commun. 6:5600 doi: 10.1038/ncomms6600 (2015).